A general thermodynamics-triggered competitive growth model to guide the synthesis of two-dimensional nonlayered materials Two-dimensional (2D) nonlayered materials have recently provoked a surge of interest due to their abundant species and attractive properties with promising applications in catalysis, nanoelectronics, and spintronics. However, their 2D anisotropic growth still faces considerable challenges and lacks systematic theoretical guidance. Here, we propose a general thermodynamics-triggered competitive growth (TTCG) model providing a multivariate quantitative criterion to predict and guide 2D nonlayered materials growth. Based on this model, we design a universal hydrate-assisted chemical vapor deposition strategy for the controllable synthesis of various 2D nonlayered transition metal oxides. Four unique phases of iron oxides with distinct topological structures have also been selectively grown. More importantly, ultra-thin oxides display high-temperature magnetic ordering and large coercivity. Mn x Fe y Co 3-x-y O 4 alloy is also demonstrated to be a promising room-temperature magnetic semiconductor. Our work sheds light on the synthesis of 2D nonlayered materials and promotes their application for room-temperature spintronic devices. Two-dimensional (2D) nonlayered materials have come under the spotlight of scientific and engineering research due to their abundant species as well as novel properties, such as enhanced surface activity [1] , anomalous thickness-dependent magnetism [2] , outstanding photodetectivity [3] , and so on, which is a crucial extension and supplement to 2D layered materials. More importantly, 2D nonlayered materials could overcome the recent dilemma faced by 2D layered magnets [4] , [5] , i.e., poor stability, low transition temperatures, and less variety. However, the controllable synthesis of 2D nonlayered materials remains an enormous challenge. Firstly, nonlayered materials are constructed with strong chemical bonds in all directions, inherently impeding 2D anisotropic growth. Secondly, they always have various phase structures and multiple components. For example, nonlayered iron oxides are polymorphic (Fe 3 O 4 , γ -Fe 2 O 3 , ε -Fe 2 O 3 , and α -Fe 2 O 3 ) with disparate properties [6] , [7] , [8] , [9] . In this regard, selective synthesis of one single-phase crystal is very challenging, not to mention the 2D growth of multi-element nonlayered materials. Thirdly, there is still a lack of general economical methods to produce high-quality 2D single crystals with desired thickness and morphology. In addition to experimental challenges, the understanding of 2D anisotropic growth mechanism for nonlayered materials is still in its infancy and desiderates a deep exploration. Unfortunately, major theoretical efforts are dedicated to investigating van der Waals (vdW) layered materials merely [10] , [11] . A generic model to interpret the growth of both layered and nonlayered materials is still missing, and quantitative models are incredibly rare. Moreover, the key driving force for forming ultra-thin 2D structures as the result of competition between vertical and lateral growth remains indistinct. The development of growth theory could not only explain the experimental phenomena but also promote the growth progress in turn. Hence, a versatile model to thoroughly comprehend 2D nonlayered material synthesis as well as the related factors is urgently desirable. Herein, we propose a general thermodynamics-triggered competitive growth (TTCG) model to provide an in-depth understanding and powerful guidance for the synthesis of 2D nonlayered materials (including oxides, chalcogens, and oxyhalides). Guided by this model, we design a universal hydrate-assisted chemical vapor deposition (HACVD) method to synthesize a library of 2D nonlayered transition metal oxide (TMO) nanoflakes (including 9 binary, 4 ternary, and even 6 alloy oxides). Moreover, phase-controllable growth of four different iron oxides can also be achieved. Raman spectra and atomic-resolution scanning transmission electron microscopy-annular dark-field (STEM-ADF) imaging confirm the composition, phase structure, and growth orientation of as-grown nanoflakes. Importantly, various oxides exhibit attractive room-temperature magnetism, the magnetic domains of which are investigated by magnetic force microscope (MFM) measurements. Furthermore, magneto-transport characterizations reveal the room-temperature magnetic semiconductor feature of Mn x Fe y Co 3-x-y O 4 alloys, making them pioneering candidates for spintronic devices. Universal model for 2D nonlayered materials growth At first, we put forward a common formula to describe the energy of a material system. As shown in Fig. 1a, we assumed all materials can be regarded as n superimposed subunits (a slab with the smallest repeating unit along the z -axis) that are interconnected to each other. The total free energy of the system ( E free ) with n superimposed subunits consists of the following parts: (1) the energy of every stacking subunit that exists alone, (2) interunit interaction, (3) edge formation energy. Hence, E free can be expressed as 
    E_free=∑_i=1^nE_iA_S-∑_i=1^n-1ε_i,i+1A_S+∑_i=1^nλ_iA_L
 (1) where E i , ε i,i +1 , λ i refer to the free energy per unit area of isolated subunit i , the interaction energy between subunit i and i + 1, and the edge energy of subunit i , respectively. A S and A L denote the surface and lateral area. Fig. 1: The thermodynamics-triggered competitive growth (TTCG) model. a Schematic illustration of \({\varepsilon }_{i,i+1}\) and \({\lambda }_{i}\) in the Eq. ( 1 ) and the representations in nonlayered and layered materials. \({\varepsilon }_{i,i+1}\) and \({\lambda }_{i}\) refer to the interaction energy per unit area between subunit i and i + 1, and the edge energy per unit area of subunit i , respectively. b Sketch map of vertical and lateral growth when a new cluster (yellow) grows with the n stacking subunits (lilac). The free energy change of vertical growth mainly comes from the interaction of subunit at the upper interface, while edge energy penalty is dominant for lateral growth. ∆ E ver and ∆ E lat represent the free energy change of vertical and lateral growth. \({\varepsilon }_{n,n+1}\) denotes the interaction energy between subunit n and n + 1. \({\lambda }_{n}\) and \({\lambda }_{B}\) represent the average edge energies of the initial structure and the new cluster, respectively. \({A}_{{s}_{B}}\) and \({A}_{{l}_{B}}\) are the basal and lateral contact areas. c The competition between \(\varepsilon\) term and \(\lambda\) term. Smaller \(\varepsilon\) term will promote lateral growth and smaller \(\lambda\) term leads to vertical growth. \({\varepsilon }_{c}\) is the circumstance correction term of the interaction energy and \({\lambda }_{c}\) is the circumstance correction term of the edge energy. d A schematic for the growth process of 2D Fe 3 O 4 nanoflakes along the [111] direction guided by the TTCG model. The intrinsic binding energy difference is not negative enough. The facilitation of H 2 O passivation (large \({\varepsilon }_{c}\) ) and mica substrate (small \({\lambda }_{c}\) ) lead to smaller ∆ E , and therefore promote the synthesis of ultrathin Fe 3 O 4 nanoflakes. e Every calculated value in the model for Fe 3 O 4 with different orientations. f Total ∆ E with and without circumstance correction terms for Fe 3 O 4 with different orientations. g Optimized structures of Fe 3 O 4 along the [111] direction without and with the H 2 O adsorption. h Total ∆ E of γ -, ε -, α -Fe 2 O 3 in different orientations with and without correction terms. Red triangles indicate the lowest energy. i Calculated values in the growth model of ZnO, MoS 2 , SmOCl, EuOCl, Fe 7 S 8 , and Cr 5 Te 8 . Full size image In layered materials, a subunit is generally represented by one slab between adjacent gaps, and weak vdW interaction plays a leading role between stacking subunits. As for nonlayered materials (Supplementary Figs. 1 – 3 ), the selection of subunit is more complex and needs to be discussed individually. More importantly, non-negligible strong covalent binding plays a part, so ε i,i +1 is relatively larger and influenced by n . 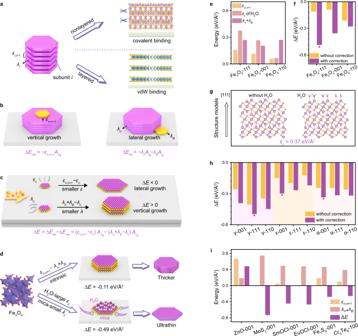Fig. 1: The thermodynamics-triggered competitive growth (TTCG) model. aSchematic illustration of\({\varepsilon }_{i,i+1}\)and\({\lambda }_{i}\)in the Eq. (1) and the representations in nonlayered and layered materials.\({\varepsilon }_{i,i+1}\)and\({\lambda }_{i}\)refer to the interaction energy per unit area between subunitiandi+ 1, and the edge energy per unit area of subuniti, respectively.bSketch map of vertical and lateral growth when a new cluster (yellow) grows with thenstacking subunits (lilac). The free energy change of vertical growth mainly comes from the interaction of subunit at the upper interface, while edge energy penalty is dominant for lateral growth. ∆Everand ∆Elatrepresent the free energy change of vertical and lateral growth.\({\varepsilon }_{n,n+1}\)denotes the interaction energy between subunitnandn+ 1.\({\lambda }_{n}\)and\({\lambda }_{B}\)represent the average edge energies of the initial structure and the new cluster, respectively.\({A}_{{s}_{B}}\)and\({A}_{{l}_{B}}\)are the basal and lateral contact areas.cThe competition between\(\varepsilon\)term and\(\lambda\)term. Smaller\(\varepsilon\)term will promote lateral growth and smaller\(\lambda\)term leads to vertical growth.\({\varepsilon }_{c}\)is the circumstance correction term of the interaction energy and\({\lambda }_{c}\)is the circumstance correction term of the edge energy.dA schematic for the growth process of 2D Fe3O4nanoflakes along the [111] direction guided by the TTCG model. The intrinsic binding energy difference is not negative enough. The facilitation of H2O passivation (large\({\varepsilon }_{c}\)) and mica substrate (small\({\lambda }_{c}\)) lead to smaller ∆E, and therefore promote the synthesis of ultrathin Fe3O4nanoflakes.eEvery calculated value in the model for Fe3O4with different orientations.fTotal ∆Ewith and without circumstance correction terms for Fe3O4with different orientations.gOptimized structures of Fe3O4along the [111] direction without and with the H2O adsorption.hTotal ∆Eofγ-,ε-,α-Fe2O3in different orientations with and without correction terms. Red triangles indicate the lowest energy.iCalculated values in the growth model of ZnO, MoS2, SmOCl, EuOCl, Fe7S8, and Cr5Te8. A detailed comparison is shown in Supplementary Table 1 . Chemical vapor deposition (CVD) method is considered as a facile route to obtain various high-quality 2D materials [12] , [13] . In the CVD growth process, we assume a new growth cluster (with the basal and lateral contact area of \({A}_{{s}_{B}}\) and \({A}_{{l}_{B}}\) , which are supposed to be equal) combines with the initial structure ( n stacking subunits) in two ways, i.e., vertically or laterally (Fig. 1b ). Based on the above analysis (more details in Supplementary Note 1 ), the free energy change of vertical growth (∆ E ver ) mainly comes from the binding force of subunit at the upper interface, while edge energy penalty is dominant for lateral growth (∆ E lat ): 
    E_ver=-ε_n,n+1A_s_B
 (2) 
    E_lat=-λ_nA_l_B-λ_BA_l_B
 (3) where λ n and λ B represent the average edge energies of the initial structure and the new cluster, respectively. The values of \({\triangle E}_{{ver}}\) and \({\triangle E}_{{lat}}\) directly reflect the growth tendency along vertical or lateral direction, so their difference (∆ E ) can be evaluated as the criterion of growth modes: 
    E= E_lat- E_ver=ε_n,n+1A_s_B-(λ_n+λ_B)A_l_B
 (4) In fact, surrounding microscopic atomic circumstances could also influence these energies in a realistic growth process, in addition to the material itself. Consequently, we introduce the circumstance correction terms ( \({\varepsilon }_{c}\) and \({\lambda }_{c}\) ) to optimize our model, and the Eq. ( 4 ) can be modified as follows: 
    E=(ε_n,n+1 - ε_c)A_s_B-(λ_n+λ_B-λ_c)A_l_B
 (5) Accordingly, lateral or vertical growth is the result of competition between \(\varepsilon\) term ( \({\varepsilon }_{n,n+1}-{\varepsilon }_{c}\) ) and \(\lambda\) term ( \({\lambda }_{n}+{\lambda }_{B}-{\lambda }_{c}\) ), which is based on thermodynamics triggering (Fig. 1c ). 2D growth (lateral growth configuration) is favored when \(\triangle E\) is negative. With respect to the intrinsic features of materials, a larger difference between \({\varepsilon }_{n,n+1}\) and \({\lambda }_{n}\) ( \({\varepsilon }_{n,n+1}\) is smaller and \({\lambda }_{n}\) is larger) will promote 2D growth. For instance, \({\varepsilon }_{n,n+1}\) is rather small in vdW materials, consistent with their monolayer growth tendency [14] , [15] . Moreover, the interface adsorption or passivation can increase \({\varepsilon }_{c}\) (by interacting with surface atoms) to decrease \(\triangle E\) and facilitate 2D growth [16] , [17] , which has not been quantitatively exhibited in previous literatures. 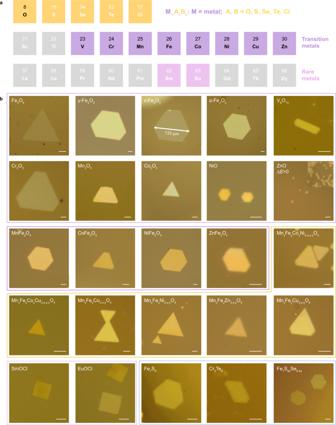Fig. 2: Synthesis of nonlayered materials guided by TTCG model. aSummary of the nonlayered materials applicable to the TTCG model. The elements highlighted in purple or pink denote transition or rare metals whose oxides, oxyhalides, or chalcogenides with nonlayered structures are demonstrated to have the potential to form 2D structures. The elements highlighted in yellow represent the available anions of nonlayered materials. The elements in black color indicate their oxides can be synthesized by our hydrate-assisted chemical vapor deposition (HACVD) method. m, a, and b are the corresponding stoichiometric numbers.bOptical images of as-grown materials. Scale bars, 5 μm. Binary, ternary, and alloy oxides are outlined in lilac, purple, and yellow colors, respectively. Rare earth oxyhalides are outlined in pink and transition metal chalcogens are marked in blue. Furthermore, substrates are also of great importance by influencing λ c , as the diffusion barrier resists edge growth [18] , which can be equivalent to an additional edge energy correction (Supplementary Table 2 ). In brief, as-proposed model provides a concrete criterion to predict and guide 2D growth, including the effect of both intrinsic materials characteristics and exterior growth conditions. Besides, it offers a quantitative way to predict the growth modes (vertically or laterally) or 2D growth difficulty based on the sign and absolute value of ∆ E . More importantly, the key growth factor is clarified by analyzing the influence of multivariate, providing powerful guidance for effective regulation of experiments. This model is applicable both to layered and especially to nonlayered materials, extending the theoretical research on 2D materials growth. Synthesis of 2D nonlayered materials guided by TTCG model TMO is a crucial class of nonlayered family with unique magnetic properties, such as topological spin states [19] , [20] , multiferroic order [21] , [22] , and Verwey transition [23] , which have held great prospects in spin filter [24] , [25] , magnetic recording [26] , magnetoelectric coupling [27] , [28] , and so on. The formation of ultrathin TMO may overcome the limitations of 2D magnets, but its controllable growth is still a grand difficulty. Therefore, we focus on TMO as the main examples to illustrate the TTCG model. 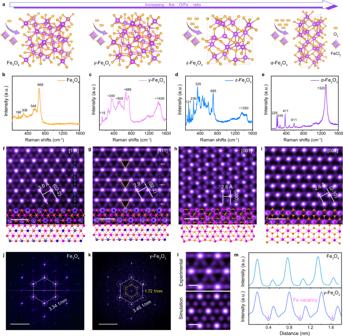Fig. 3: Structural characterizations of four iron oxides with different structures. aStructures of four iron oxides. With increasing the O/Fe ratio, Fe3O4,γ-Fe2O3,ε-Fe2O3, andα-Fe2O3in different structures can be obtained, respectively. Double spheres represent O2molecules; octahedrons represent FeCl2molecules; the orange and purple spheres denote O and Fe atoms, respectively. Dashed rectangles represent unit cells.b–eRaman vibration modes are indexed to Fe3O4(b),γ-Fe2O3(c),ε-Fe2O3(d), andα-Fe2O3(e), respectively. Raman spectra of four iron oxides are totally different, and the main peaks are indicated in the figures.f–iTop-view scanning transmission electron microscopy-annular dark-field (STEM-ADF) images of Fe3O4(f),γ-Fe2O3(g),ε-Fe2O3(h), andα-Fe2O3(i), respectively, inserted with projected atomic models. The periodic yellow triangles indicate ordered Fe octahedral vacancies. The orange, purple, and blue spheres represent O, octahedral Fe, and tetrahedral Fe atoms, respectively.j,kThe corresponding fast Fourier transform (FFT) patterns of Fe3O4(j) andγ-Fe2O3(k) along the [111] direction.lThe enlarged STEM image ofγ-Fe2O3and its corresponding simulated image.mThe corresponding intensity line profiles from Fe3O4andγ-Fe2O3. The arrows indicate Fe vacancies. Scale bars:f–i0.5 nm;j,k1/5 nm;l0.2 nm. Cubic Fe 3 O 4 is taken as a representative example, because various oxides have similar structures (Supplementary Table 3 ). The intrinsic energy difference between \({\varepsilon }_{n,n+1}\) and \({\lambda }_{n}\) + \({\lambda }_{B}\) along diverse orientations is not negative enough (Fig. 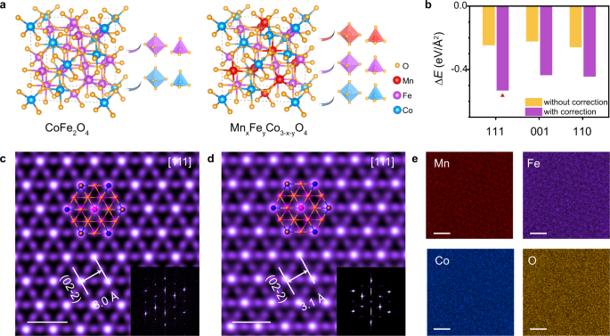Fig. 4: TTCG model for multi-element oxides. aStructure models of CoFe2O4and MnxFeyCo3-x-yO4. Metal ions occupy the centers of tetrahedrons or octahedrons sites surrounded by oxygen atoms. Dashed rectangles represent unit cells.bTotal ∆Ewith and without circumstance correction terms for CoFe2O4with different orientations based on the TTCG model. Red triangles indicate the lowest energy.c,dTop-view STEM-ADF images of CoFe2O4(c) and MnxFeyCo3-x-yO4(d) nanoflakes, inserted with corresponding projected atomic models along the [111] orientation. The orange, purple, and blue spheres represent O atoms, octahedral sites, and tetrahedral sites, respectively. Inset shows the corresponding FFT pattern, indicating the [111] orientation.eEnergy-dispersive X-ray spectroscopy (EDS) elemental mapping images of ultrathin MnxFeyCo3-x-yO4alloy. Scale bars:c,d0.5 nm;e1 nm. 1d–f , and Supplementary Table 4 ), so the inherent 2D growth is thermodynamically challenging. According to Eq. ( 5 ), increasing \({\varepsilon }_{{{{{{\rm{c}}}}}}}\) to reduce \(\varepsilon\) term is an effective approach for promoting lateral growth. Considering the surface metal atoms (Supplementary Fig. 1e ), adsorption of polar water molecules is found to significantly influence \({\varepsilon }_{c}\) (Fig. 1e and Supplementary Table 4 ). For instance, \({\varepsilon }_{c}\) of water is as large as 0.37 eV/Å 2 for Fe 3 O 4 along the [111] direction (Fig. 1g ). Besides, enhancing λ term is another way to decrease ∆ E , so mica with smaller diffusion barrier energy (i.e., smaller \({\lambda }_{c}\) ) is considered as a better growth substrate (Supplementary Table 2 ). As a result, [111] direction is predicted to be the preferred growth orientation with the lowest ∆ E of −0.49 eV/Å 2 (Fig. 1f ), which is more negative at this time to favor 2D growth (Fig. 1d ). In addition to Fe 3 O 4 , other Fe-based oxides are also predicted to have a good chance to form 2D nanoflakes under the action of water and mica (Fig. 1h ), which are thoroughly discussed in the next section. Based on these theoretical analyses, a HACVD growth strategy was designed to produce TMO nanoflakes on mica substrate. Hydrate is adopted to deliver a controlled amount of water vapor at a preset time to promote 2D growth. Transition metal chloride with lower melting points and oxygen were employed as precursors. Several ultra-thin 2D oxides can be synthesized by this method, including iron oxides, V 6 O 13 , Cr 2 O 3 , Mn 3 O 4 , Co 3 O 4 , and NiO nanoflakes, as indicated in Fig. 2 . However, ZnO nanorods are obtained instead of nanoflakes. The calculated Δ E of ZnO based on the model is positive with 0.48 eV/Å 2 (Fig. 1i ), so it is unfavorable for 2D growth, which is in good agreement with the experiment. In addition, because chlorides are employed as precursors whose melting points are close among different metals, the HACVD method can also be extended to multi-element oxides. The details are discussed in the following. Four types of ternary ferrite MFe 2 O 4 (M = Mn, Co, Ni, Zn) and six kinds of alloy oxides (quaternary and quinary oxides) are obtained. The thickness of these 2D oxides can be down to several nanometers (Supplementary Fig. 4 ), thanks to the use of H 2 O and mica under the guidance of the model. Fig. 2: Synthesis of nonlayered materials guided by TTCG model. a Summary of the nonlayered materials applicable to the TTCG model. The elements highlighted in purple or pink denote transition or rare metals whose oxides, oxyhalides, or chalcogenides with nonlayered structures are demonstrated to have the potential to form 2D structures. The elements highlighted in yellow represent the available anions of nonlayered materials. The elements in black color indicate their oxides can be synthesized by our hydrate-assisted chemical vapor deposition (HACVD) method. m, a, and b are the corresponding stoichiometric numbers. b Optical images of as-grown materials. Scale bars, 5 μm. Binary, ternary, and alloy oxides are outlined in lilac, purple, and yellow colors, respectively. Rare earth oxyhalides are outlined in pink and transition metal chalcogens are marked in blue. Full size image In addition to oxides, we also apply this model to other layered and nonlayered materials (Fig. 1i and Supplementary Table 4 ). As is well-known, layered MoS 2 is inclined to grow into 2D monolayer [29] , [30] , in line with the calculated ∆ E (as low as −0.73 eV/Å 2 ). Besides, some nonlayered rare-earth metal oxyhalides (EuOCl, SmOCl) and transition metal chalcogens (Cr 5 Te 8 , Fe 7 S 8 , and In 2 Se 3 ) are also predicted to possess intrinsic negative ∆ E with a good potential to form 2D nanoflakes, which is experimentally verified by CVD method as well (Fig. 2b ). The synthesis of these binary and even multi-element nonlayered oxides, chalcogens, and oxyhalides offer credible evidence for the universality and feasibility of our growth model. Demonstration of TTCG model in oxides of distinct structures Notably, iron oxides possess diversified structures or phases in different space groups (Fig. 3a and Supplementary Table 3 ). Based on the TTCG model (Fig. 1h and Supplementary Table 4 ), cubic γ -Fe 2 O 3 , orthogonal ε -Fe 2 O 3 , and trigonal α -Fe 2 O 3 also possess relatively negative ∆ E (−0.50 eV/Å 2 , −0.30 eV/Å 2 , −0.34 eV/Å 2 ), after introducing the correction term of water ( \({\varepsilon }_{c}\) ), indicating that they all have the potential to form 2D structures with the predicted orientation along the [111], [001], and [001] direction, respectively. Fig. 3: Structural characterizations of four iron oxides with different structures. a Structures of four iron oxides. With increasing the O/Fe ratio, Fe 3 O 4 , γ -Fe 2 O 3 , ε -Fe 2 O 3 , and α -Fe 2 O 3 in different structures can be obtained, respectively. Double spheres represent O 2 molecules; octahedrons represent FeCl 2 molecules; the orange and purple spheres denote O and Fe atoms, respectively. Dashed rectangles represent unit cells. b – e Raman vibration modes are indexed to Fe 3 O 4 ( b ), γ -Fe 2 O 3 ( c ), ε -Fe 2 O 3 ( d ), and α -Fe 2 O 3 ( e ), respectively. Raman spectra of four iron oxides are totally different, and the main peaks are indicated in the figures. f – i Top-view scanning transmission electron microscopy-annular dark-field (STEM-ADF) images of Fe 3 O 4 ( f ), γ -Fe 2 O 3 ( g ), ε -Fe 2 O 3 ( h ), and α -Fe 2 O 3 ( i ), respectively, inserted with projected atomic models. The periodic yellow triangles indicate ordered Fe octahedral vacancies. The orange, purple, and blue spheres represent O, octahedral Fe, and tetrahedral Fe atoms, respectively. j , k The corresponding fast Fourier transform (FFT) patterns of Fe 3 O 4 ( j ) and γ -Fe 2 O 3 ( k ) along the [111] direction. l The enlarged STEM image of γ -Fe 2 O 3 and its corresponding simulated image. m The corresponding intensity line profiles from Fe 3 O 4 and γ -Fe 2 O 3 . The arrows indicate Fe vacancies. Scale bars: f – i 0.5 nm; j , k 1/5 nm; l 0.2 nm. Full size image Indeed, four kinds of ultrathin iron oxides nanoflakes with distinct topology structures can be synthesized by the HACVD method. The thickness can also be regulated by changing the mass of hydrate (Supplementary Fig. 5 ), illustrating the importance of \({\varepsilon }_{c}\) by water for promoting 2D growth. These results verify the reliability of the prediction results of the TTCG model. Moreover, the phase-controllable growth can be realized as well, which is found to strongly depend on the O/Fe ratio in HACVD process (Supplementary Fig. 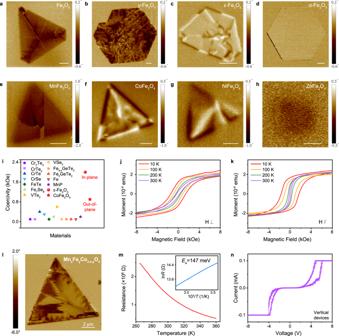Fig. 5: Room-temperature magnetism and electrical properties of oxides. a–hMagnetic force microscope (MFM) phase images of Fe3O4(7.8 nm),γ-Fe2O3(7.3 nm),ε-Fe2O3(10 nm),α-Fe2O3(27 nm), MnFe2O4(20 nm), CoFe2O4(18 nm), NiFe2O4(15 nm), ZnFe2O4(29 nm), respectively. Scale bars:a–d, 2 μm;e–h, 1 μm.iComparison of coercivity at 200 K inε-Fe2O3and CoFe2O4with other 2D magnets.jMagnetic hysteresis of MnxFeyCo3-x-yO4alloy with magnetic field perpendicular to the substrate.kMagnetic hysteresis of MnxFeyCo3-x-yO4alloy with magnetic field parallel to the substrate.lRoom-temperature MFM phase image of MnxFeyCo3-x-yO4alloy (16.2 nm).mTemperature-dependent longitudinal resistance of MnxFeyCo3-x-yO4alloy from 260 K to 360 K. Inset: Fitted curves by Arrhenius equation, indicating the activation energy of 147 meV.nCurrent–voltage characteristic sweep of the vertical device under ambient conditions. The current compliance is 0.1 mA. 6 and Supplementary Table 5 ). As exhibited in Fig. 3b–e and Supplementary Table 6 , four kinds of iron oxides exhibit entirely different Raman vibration modes, making them easily distinguished [9] , [31] , [32] , [33] , [34] , [35] , [36] . To further study the atomic structure and growth orientation of the iron oxides, atomic-resolution STEM-ADF imaging was employed to reveal the structures of diverse phases. Fe atoms can be directly distinguished from O atoms by the bright contrast. STEM-ADF images of Fe 3 O 4 and γ -Fe 2 O 3 (Fig. 3f, g ) reveal a periodic bright and dark spots arrangement, i.e., each bright atomic column is surrounded by dark hexagon-arranged atomic columns, which is the hallmark of approximately isostructural cubic Fe 3 O 4 and γ -Fe 2 O 3 . Based on their structures, the bright contrast is mainly related to the quantity of Fe atoms rather than the atomic number. Specifically, the light dots are atomic columns containing both tetrahedral and octahedral sites, while the dark dots only contain octahedral sites, consistent with the projected atomic structure along [111] direction. Intriguingly, the fast Fourier transform (FFT) image of γ -Fe 2 O 3 (Fig. 3k ) exhibits a series of periodic superspots (marked by the yellow circles), which is absent in Fe 3 O 4 (Fig. 3j ). The superspots are originated from ordered Fe octahedral vacancies, labeled in Fig. 3g and Fig. 3m , in line with the simulated images (Fig. 3l ). Although the presence of ordered vacancies in γ -Fe 2 O 3 crystals was known from previous works [37] , [38] , the STEM image presented here provides the real-space evidence for octahedral vacancies in γ -Fe 2 O 3 . The structures of orthorhombic ε -Fe 2 O 3 and trigonal α -Fe 2 O 3 are also verified by the consistency of the experimental images and the atomic models along [001] zone axes, respectively (Fig. 3h, i ). Notably, the observed crystal orientations of STEM are all consistent with the predictions of the model. The successful growth of 2D nonlayered iron oxides with four different structures demonstrates TTCG model is not limited by the crystal structures, illustrating the universality of our model from another perspective. It is worth noting that although Fe 3 O 4 , γ -Fe 2 O 3 , and ε -Fe 2 O 3 have been prepared by CVD method previously [34] , [35] , [36] , the key factor of phase-controllable growth is revealed here. The sizes and qualities of our samples also exceeded the preceding reports (compared in Supplementary Table 7 ). Demonstration of TTCG model in multi-element oxides TTCG model can also be applied to multi-element oxides. Multi-element oxides crystallize into similar spinel-type structures, where metal ions occupy the centers of tetrahedrons or octahedrons sites surrounded by oxygen atoms (Fig. 4a ). Taking CoFe 2 O 4 as an example, the adsorption of water significantly influences \({\varepsilon }_{c}\) (0.29 eV/Å 2 as shown in Supplementary Table 4 ), and it is predicted to have a great potential to form 2D nanoflakes with a negative ∆ E of −0.53 eV/Å 2 along the [111] direction (Fig. 4b ). The X-ray diffraction (XRD) pattern of CoFe 2 O 4 (Supplementary Fig. 7 ) can be indexed to the cubic structure with lattice parameters of a = b = c = 8.39 Å, and nanoflakes are well aligned with the [111] direction, in accord with the prediction by TTCG model. Fig. 4: TTCG model for multi-element oxides. a Structure models of CoFe 2 O 4 and Mn x Fe y Co 3-x-y O 4 . Metal ions occupy the centers of tetrahedrons or octahedrons sites surrounded by oxygen atoms. Dashed rectangles represent unit cells. b Total ∆ E with and without circumstance correction terms for CoFe 2 O 4 with different orientations based on the TTCG model. Red triangles indicate the lowest energy. c , d Top-view STEM-ADF images of CoFe 2 O 4 ( c ) and Mn x Fe y Co 3-x-y O 4 ( d ) nanoflakes, inserted with corresponding projected atomic models along the [111] orientation. The orange, purple, and blue spheres represent O atoms, octahedral sites, and tetrahedral sites, respectively. Inset shows the corresponding FFT pattern, indicating the [111] orientation. e Energy-dispersive X-ray spectroscopy (EDS) elemental mapping images of ultrathin Mn x Fe y Co 3-x-y O 4 alloy. Scale bars: c , d 0.5 nm; e 1 nm. Full size image Figure 4c–e shows the STEM-ADF and energy-dispersive X-ray spectroscopy (EDS) elemental mapping images of ultrathin CoFe 2 O 4 and Mn x Fe y Co 3-x-y O 4 alloy, respectively. The STEM images and FFT patterns exhibit perfect hexagonally arranged lattice fringes and high-quality single-crystalline phases with the [111] orientation (Fig. 4c, d ), the same as the predicted orientation by the model (Fig. 4b ). Due to the complicated atoms distribution of spinel-type structure and the similar atomic number of Co/Fe/Mn, the actual positions of different elements are difficult to be discriminated. In addition, the nanoscale EDS elemental mappings confirm that Mn, Fe, Co, and O are uniformly distributed throughout the entire crystal (Fig. 4e and Supplementary Fig. 7c ). Cross-section STEM (Supplementary Fig. 8 ) results show that the surface of CoFe 2 O 4 is likely to be passivated by the hydroxyl group, which further demonstrates the significant role of \({\varepsilon }_{c}\) (by water) for promoting 2D growth and is in line with the model as well. The successful growth of multi-element oxides illustrates that TTCG model is not limited by chemical composition and can be applied to guide multi-element nonlayered materials growth. The detailed characterizations of other oxides and oxyhalides or chalcogens are provided in Supplementary Figs. 9 – 22 . Magnetic properties of oxides The successful synthesis of various TMO nanoflakes under the guidance of TTCG model has also enabled us to explore their unique properties. 2D TMO nanoflakes possess rich magnetic properties, ranging from antiferromagnets to soft magnets and hard magnets, which are characterized in Supplementary Figs. 23 – 25 and summarized in Supplementary Table 8 . Importantly, most of them exhibit fascinating room-temperature magnetic ordering with high stability. In principle, oxides are more stable against air and water corrosion than chalcogens and chlorides. As exhibited in Supplementary Fig. 26 , the surface topography of iron oxides shows no obvious oxidation after exposure to air for three months. To further demonstrate the room-temperature magnetism of 2D oxides nanoflakes, we measured their magnetic domain structure via MFM. As indicated in Fig. 5a–d and Supplementary Figs. 27–29 , four iron oxides exhibit distinct domain patterns, confirming the realization of phase-controllable growth by our HACVD method from another perspective: Fe 3 O 4 possesses out-of-plane triangular magnetic domains, and γ -Fe 2 O 3 shows out-of-plane dendritic-like magnetic domains. Differently, flux-closure magnetic domains are imaged in ε -Fe 2 O 3 . The MFM phase contrast between ε -Fe 2 O 3 and substrates is weaker, and the magnetic signal across the line profile exhibits double peaks (Supplementary Fig. 28 ), indicating the in-plane magnetism of ε -Fe 2 O 3 . However, it is hard to discern the magnetic signals of α -Fe 2 O 3 , attributed to its antiferromagnetic behavior [19] . Moreover, the observation of magnetic domain signals in ultrathin ferrites (Fig. 5e–h ) also provides evidence for the existence of room-temperature magnetism in ternary oxides nanoflakes. Different compositions have disparate magnetic signal intensity and domain states. Fig. 5: Room-temperature magnetism and electrical properties of oxides. a – h Magnetic force microscope (MFM) phase images of Fe 3 O 4 (7.8 nm), γ -Fe 2 O 3 (7.3 nm), ε -Fe 2 O 3 (10 nm), α -Fe 2 O 3 (27 nm), MnFe 2 O 4 (20 nm), CoFe 2 O 4 (18 nm), NiFe 2 O 4 (15 nm), ZnFe 2 O 4 (29 nm), respectively. Scale bars: a – d , 2 μm; e – h , 1 μm. i Comparison of coercivity at 200 K in ε -Fe 2 O 3 and CoFe 2 O 4 with other 2D magnets. j Magnetic hysteresis of Mn x Fe y Co 3-x-y O 4 alloy with magnetic field perpendicular to the substrate. k Magnetic hysteresis of Mn x Fe y Co 3-x-y O 4 alloy with magnetic field parallel to the substrate. l Room-temperature MFM phase image of Mn x Fe y Co 3-x-y O 4 alloy (16.2 nm). m Temperature-dependent longitudinal resistance of Mn x Fe y Co 3-x-y O 4 alloy from 260 K to 360 K. Inset: Fitted curves by Arrhenius equation, indicating the activation energy of 147 meV. n Current–voltage characteristic sweep of the vertical device under ambient conditions. The current compliance is 0.1 mA. Full size image It is worth noting that ε -Fe 2 O 3 and CoFe 2 O 4 are both hard magnets, the coercivity of which is larger than most reported 2D magnets [5] , [39] , [40] , [41] , [42] , [43] , [44] , [45] , [46] , [47] , [48] , [49] , as shown in Fig. 5i and Supplementary Fig. 30 . The discovered high-temperature 2D magnets are rare, let alone one owning large coercivity above 200 K, which has great application prospects in high-density magnetic recording and storage. As for ε -Fe 2 O 3 , the coercivity is ~2000 Oe in the in-plane direction. Moreover, out-of-plane coercivity of CoFe 2 O 4 is determined to be ~900 Oe. The thickness-dependent magnetic properties of CoFe 2 O 4 are investigated by reflection magnetic circular dichroism (RMCD) and MFM measurements in Supplementary Fig. 31 . With reducing the thickness, the magnetism becomes weaker, the coercivity decreases, and multi-domain structure gets more sophisticated. In addition, alloying can further extend the magnetic material family. As depicted in Fig. 5j, k , obvious hysteresis was observed in Mn x Fe y Co 3-x-y O 4 nanoflakes regardless of applying a perpendicular or parallel magnetic field, showing the room-temperature magnetic ordering and large coercivity. Temperature-dependent magnetization curves illustrate the ferrimagnetic behavior of Mn x Fe y Co 3-x-y O 4 alloy (Supplementary Fig. 32 ). The multi-domain magnetic states in MFM image further demonstrate the room-temperature magnetism of an individual Mn x Fe y Co 3-x-y O 4 nanoflake, which is well maintained with thickness even down to 3.5 nm (Fig. 5l and Supplementary Fig. 33 ). To explore the electrical properties, devices are fabricated on Mn x Fe y Co 3-x-y O 4 nanoflakes transferred to SiO 2 /Si substrate (Supplementary Fig. 34 ). The anomalous Hall effect and butterfly-shaped hysteresis behavior of magneto-resistance curves (Supplementary Fig. 35 ) also indicate the appearance of magnetic ordering in Mn x Fe y Co 3-x-y O 4 . Figure 5m displays the temperature-dependent resistance ( \(R\) ) which increases gradually with decreasing temperatures, declaring the typical semiconductor feature. By fitting the Arrhenius equation ( \({{{{{\rm{ln}}}}}}{R}={{{{\mathrm{ln}}}}}{R}_{0}+{E}_{a}/{k}_{B}T\) , where \({k}_{B}\) is Boltzmann constant, T is the temperature, and \({R}_{0}\) is the fitting parameter), the activation energy ( \({E}_{a}\) ) is estimated to be 147 meV. Resistive switching behavior is also observed in the vertical devices of Mn x Fe y Co 3-x-y O 4 alloy (Fig. 5n and Supplementary Fig. 36 ). When the voltage sweeps back and forth, the current does not overlap, illustrating the semiconductor behavior as well. In summary, we have proposed a TTCG model to get a new insight into the synthesis of 2D materials. It offers a multivariate quantitative criterion, which can not only predict the growth modes but also provide powerful guidance for experiments. For instance, specific crystal orientation, the adoption of water vapor, and the selection of substrate are considered to promote the 2D anisotropic growth of oxides. In addition, this model is not limited by crystal structures or element compositions, which is generalized both to layered and especially to nonlayered materials (including oxides, chalcogens, and oxyhalides), promoting the theoretical research and chemical synthesis of 2D materials. Guided by the model, we design a universal HACVD strategy to synthesize a family of 2D nonlayered TMO nanoflakes, including 9 binary, 4 ternary, and 6 alloy oxides. Moreover, phase-controllable growth of Fe-based oxides (Fe 3 O 4 and γ -, ε -, α -Fe 2 O 3 ) can also be achieved. Importantly, the attracting room-temperature magnetic ordering, high stability, rich magnetic domain structure, larger coercivity, and semiconductivity of as-synthesized oxides nanoflakes can further expand the family of 2D magnets, and provide alternative platforms for pioneering applications in room-temperature magnetoelectronic or spintronic devices. Synthesis of oxides 2D iron oxides were synthesized on mica substrates via hydrate-assisted CVD method. The reaction was conducted in a one-inch quartz tube heated by a three-zone furnace (Lindberg/Blue M). ~800 mg CaSO 4 ·2H 2 O powder (99.5%, Alfa Aesar) was put at the upstream as the water source, the temperature of which is set at ~130 °C. ~15 mg Ferrous chloride (99.5%, Alfa Aesar) was placed in an alumina boat downstream. Freshly cleaved fluorophlogopite mica (Taiyuan Fluorphlogopite Mica Company Ltd, 10 × 10 × 0.2 mm) is used as the substrate and put 1–3 cm away from ferrous chloride. Prior to the growth, the furnace was purged by 400 sccm high-purity Ar gas for 15 min to remove the residual air. Then, 100 sccm Ar were inlet as the carrier gas during the whole growth process. O 2 was introduced into the CVD system at the beginning of heating for different times to synthesize different phases of iron oxides. The growth zone of ferrous chloride was heated to 550–700 °C for 20 min, and kept for another 10 min for growth. As for other oxides, corresponding metal chlorides are employed, and the growth conditions are similar with iron oxides. The detailed synthesis recipes of transition-metal-based oxides are provided in Supplementary Table 9 . Synthesis of oxyhalide 50 mg EuCl 3 ·6H 2 O or SmCl 3 ·6H 2 O (98%, Alfa Aesar) and 20 mg NaCl were mixed together in an alumina boat where the temperature is set at 900 °C. Mica was placed just over the precursors with the growth time of 20 min. 20 sccm Ar was used as the carrier gas to grow EuOCl or SmOCl. Synthesis of chalcogens 20 mg CrCl 3 (98%, Alfa Aesar) and 50 mg Te (99.9%, Alfa Aesar) powders were mixed together to synthesize Cr 5 Te 8 . Precursors were placed in a quartz boat at 700 °C with a mica substrate placed face-down. Before heating, the CVD system was evacuated and filled with Ar three times to remove oxygen and moisture. Then, mixed gases of 5 sccm H 2 and 100 sccm Ar were introduced for growth. Once the reaction ended, the furnace was moved away for rapid cooling. Besides, FeCl 2 (Alfa Aesar, 99.5%) and S (Alfa Aesar, 99.5%) powder were used as the Fe and S source to synthesize Fe 7 S 8 . 100 mg S powder was placed in the first heating zone at 130 °C, and 20 mg FeCl 2 was placed in an alumina boat in the third heating zone at 560 °C. Mica was put 1 cm downstream away from FeCl 2 . Before heating, the CVD system was evacuated and filled with Ar three times to remove oxygen and moisture. 10 sccm H 2 and 100 sccm Ar were introduced and the heating time is set at ~10 min. Characterizations Optical images were characterized by Nexcope NM910 microscope. Atomic force microscope (Bruker, Dimension Icon) was employed to measure thicknesses, and MFM is conducted by the magnetic force modes with magnetic tips. EDS mapping (FEI, Tecnai F30) was used to analyze element compositions. Raman spectra were collected by Horiba, XploRA PLUS with excitation light of ~532 nm. Magnetism was characterized by the physical property measurement system (DynaCool, Quantum Design) equipped with vibrating sample magnetometry. The atomic structures of ferrites were characterized by a cold-field emission transmission electron microscope (JEOL ARM200F) operating at 200 kV. The convergent semi-angle for the incident probe was set about 30 mrad. The collection angle of the ADF images ranges from 81 to 228 mrad. Device fabrication and electrical transport measurement Oxides nanoflakes were transferred from mica to Si/SiO 2 substrates via poly(methyl methacrylate)-assisted method. Then, devices were defined by standard e-beam lithography (FEI NanoSEM). 5 nm Ti and 60 nm Au were deposited by e-beam evaporation to be adopted as the contact electrodes. For vertical devices, 20 nm Au was used for bottom electrodes. Two-electrode testings were carried out on a probe station (Lakeshore TTP4) equipped with a vacuum pump and Keithley 4200 semiconductor analyzer. Magneto-transport measurements were conducted by four-probe electrical measurements in a commercial physical property measurement system (DynaCool, Quantum Design) with magnetic field vertical to the sample and temperature from 260 K to 360 K. Density functional theory calculations The geometrical optimizations were performed by DFT based on Perdew-Burke-Ernzerhof generalized gradient approximation (PBE-GGA) functional [50] , implemented in Vienna Ab-initio Simulation Package (VASP) [51] . The electronic properties were described by the projector augmented wave (PAW) potentials with a kinetic energy cutoff of 500 eV for planewave basis set, as confirmed by a convergence test [52] . The valence electron configurations for Cr (3 p 6 3 d 5 4 s 1 ), Fe (3 p 6 3 d 6 4 s 2 ), Co (3 d 7 4 s 2 ), Zn (3 d 10 4 s 2 ), Eu (4 f 7 5 s 2 5 p 6 6 s 2 ), Sm (4 f 6 5 p 6 6 s 2 ), O (2 s 2 2 p 4 ), S (3 s 2 3 p 4 ), Te (5 s 2 5 p 4 ), Cl (3 s 2 3 p 5 ), and H (1 s 1 ) were employed. The first Brillouin zone is represented by a Γ-point-centered Monkhorst–Pack k - mesh [53] with a grid density of \(2{\pi} \times 0.02\) Å −1 along each dimension. The strong correlation in the 3d orbitals of Fe, Co, Cr atoms are treated by including an on-site Coulomb interaction of \(U=4.0,3.3,3.5\) eV [54] , respectively. The non-local van der Waals (vdW) interactions were corrected with the Grimme’s zero damping DFT-D3 method [55] . The dipole-dipole interaction corrections in the z axis were incorporated [56] . The tolerance of 1.0 × 10 −5 eV for self-consistent-field (SCF) iteration was set, and the atoms of subunit slabs were allowed to be fully relaxed until all the force components decreased below 0.02 eV/Å, without any symmetry constraints.